Transforming moiré blisters into geometric graphene nano-bubbles Strain engineering has been proposed as an alternative method for manipulating the electronic properties of graphene. However, the bottleneck for strain engineering in graphene has been the ability to control such strain patterns at the nanoscale. Here we show that high level of control can be accomplished by chemically modifying the adherence of graphene on metal. Using scanning tunnelling microscopy, the shape evolution of graphene Moiré blisters towards geometrically well-defined graphene bubbles was studied during the controlled, sub-layer oxidation of the ruthenium substrate. Understanding the dynamics of the oxidation process and defects generation on the Ru substrate allows us to control the size, shape and the density of the bubbles and its associated pseudo-magnetism. We also show that a modification of the same procedure can be used to create antidots in graphene by catalytic reaction of the same nanobubbles. Graphene is a semimetal, not a semiconductor and as such the current flow in graphene-based devices cannot be completely switched off [1] , [2] , [3] , [4] , [5] . This is a large limitation for the use of graphene in digital electronics [6] , [7] . One strategy for opening the gap is the coupling of Dirac particles in graphene to strain via pseudo-magnetic fields, creating electrodynamics that is purely geometrical and that depends only on the local deformations of the honeycomb lattice [8] , [9] . However, a uniform spectral gap cannot be induced in graphene by an arbitrary strain field. The relationship between a strain texture and its associated pseudo-magnetic field pattern is not trivial and only specific strain configurations of triangular symmetry are capable of producing uniform pseudo-magnetic fields and electronic gaps [9] , [10] . It was demonstrated very recently by one report that graphene nanobubbles (GNB) can exhibit large pseudo-magnetic fields of the order of 300T at room temperature [9] . However, the detailed mechanism of how GNB arises on a perfect graphene sheet is still an open question. At present, a systematic approach towards the fabrication of strained nanostructures on graphene with precise control of shape and size is lacking. A buckling instability exists on graphene grown on Ru(0001) owing to the compressive strain between lattice-mismatched Ru and graphene, which gives rise to periodic blistering (Moiré humps) of graphene [11] , [12] , [13] , [14] , [15] . One inspiration we derived by examining the periodic blisters on the Moiré superlattice is the remarkable resemblance of these blisters to an ordered array of nano-bubbles ( Figs 1a–c, 2a ). The undulating Moiré valleys and humps consist of graphene domains that are attached to, or lifted off, the Ru substrate, respectively [11] , [12] , [13] , [14] , [15] , [16] . An interesting question is whether isolated pockets of these blisters can be expanded into bigger bubbles with larger internal strains. We hypothesized that, if the graphene can be delaminated from the valley regions in a localized manner, the hump regions can be expanded to form a bubble to accommodate the stress [17] ( Fig. 2 ) arising from the delamination process. 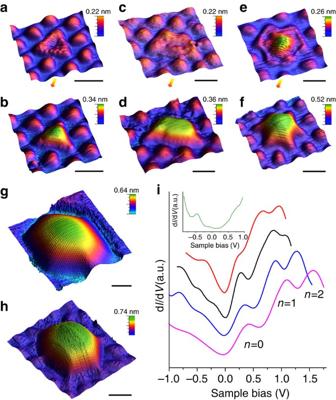Figure 1: Three-dimensional STM images of series of GNBs and their corresponding dI/dVspectra. (a–h), The coalescence of graphene blisters to form triangular, trapezoidal, and hexagonal GNBs. (i), Representative dI/dVspectra of the GNBs (100 K) in (b) (red line), (f) (blue line), (g) (black line), (h) (magenta line). Inset of i: dI/dVspectrum collected on Moiré blisters. The scale bars in (a–f) and (g–h) are 3 nm and 4 nm, respectively. Tunnelling parameters (a-h)V=0.2 V,I=0.4 nA. Figure 1: Three-dimensional STM images of series of GNBs and their corresponding d I /d V spectra. ( a – h ), The coalescence of graphene blisters to form triangular, trapezoidal, and hexagonal GNBs. ( i ), Representative d I /d V spectra of the GNBs (100 K) in ( b ) (red line), ( f ) (blue line), ( g ) (black line), ( h ) (magenta line). Inset of i: d I/ d V spectrum collected on Moiré blisters. The scale bars in ( a – f ) and ( g – h ) are 3 nm and 4 nm, respectively. Tunnelling parameters ( a - h ) V =0.2 V, I =0.4 nA. 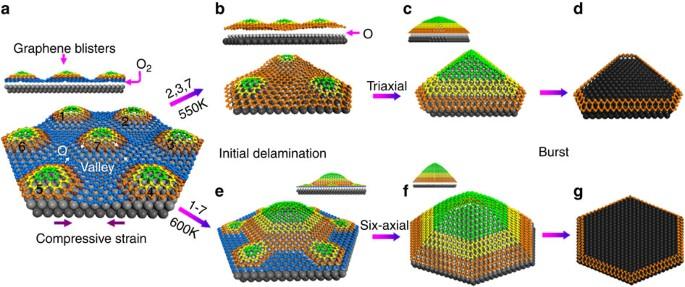Figure 2: Formation of triangular and hexagonal GNB-derived from the basic building blocks. (a) Graphene blisters are formed due to the uniform compressive strain associated with the lattice-mismatched ruthenium and graphene. The initial delamination by intercalation of O is along the two adjacent blisters as indicated by white arrows. The formation of (b–d), triangular GNB at 550 K and (e–g), hexagonal GNB at 600 K and the generation of their corresponding antidots after the GNB 'burst'. Full size image Figure 2: Formation of triangular and hexagonal GNB-derived from the basic building blocks. ( a ) Graphene blisters are formed due to the uniform compressive strain associated with the lattice-mismatched ruthenium and graphene. The initial delamination by intercalation of O is along the two adjacent blisters as indicated by white arrows. The formation of ( b–d ), triangular GNB at 550 K and ( e – g ), hexagonal GNB at 600 K and the generation of their corresponding antidots after the GNB 'burst'. Full size image In this Article, we demonstrate that oxygen intercalation at elevated temperature affects the electronic coupling between the metal substrate and graphene. At high temperatures and oxygen pressure, macroscopic regions of graphene can be delaminated from oxidized Ru(0001) [18] , [19] . O 2 molecules can diffuse through step edges and surface defects [20] and permeate between graphene and ruthenium through the hump regions of the Moiré structures. Our key idea is to oxidize only microscopic domains without ripping extended regions of graphene from ruthenium substrate. In this regard, we grew a layer of graphene on Ru(0001), and then carried out controlled oxidation of the ruthenium substrate. The evolution in the morphology of the periodic blisters during the oxidative delamination was followed using a scanning tunnelling microscope (STM). The convolution of Moiré blisters to geometric bubbles After dosing 90 Langmuir (L) of O 2 gas at 550 K, we observed that nanobubbles started to break out at random sites on the graphene. Using STM, we captured the transformation of the surface blisters as they convoluted into geometric GNBs ( Fig. 1a–f and Supplementary Fig. S1 ). The smallest GNB we observed has a triangular geometry and is directly inherited from a basic unit cell in the periodic blisters with its side dimension defined by the lattice constant of Moiré pattern, that is, 30 Å. It follows that, during the initial stages of the oxidation reaction, 90% of the GNBs are triangles and have a uniform size distribution, as shown below. The geometric centre of the triangular GNB coincides with the centre of valley region between three nearest-neighbour blisters ( Figs 1a–b and 2a–c ). The intercalated O atoms act as 'scissors' to cut the C–Ru bonds, allowing three blisters to convolute into a triangular GNB. Coalescence of 5 and 7 blisters gives rise to the trapezoid-shaped and hexagon-shaped GNBs, respectively, as indicated in Fig. 1c–f . The trapezoid nanobubbles occur with a lower frequency on the surface because it involves the sintering of 5 blisters, and the final structure has a lower symmetry compared with the triangular or hexagonal nanobubbles. From the temperature dependence of the shape evolution of the nanobubbles during the oxygenation reaction, we can infer that the nanobubble is a kinetically driven product. The total interaction energy (adhesion and bending energy) per Moiré unit cell for 288 carbon atoms is calculated to be −11.6 eV (0.4 eV per C) [13] . To produce larger sized nanobubbles, larger activation energies are involved, because larger regions have to be delaminated. For example, the production of a hexagonal bubble requires the delamination of 6 'valley' regions, which is equivalent to three Moiré units. The energy cost of 34.8 eV (11.6 eV×3) to detach a hexagonal patch of graphene from the metal substrate is offset in part by the elastic energy gain due to the strain relaxation in decoupled regions. In contrast, the energy cost to produce a triangular GNB is lower at 5.8 eV (11.6 eV×1/2), because only 1 valley region needs to be delaminated. This explains why there is a temperature dependence in the morphology of the GNBs. Using the same oxygen dosage and annealing time, triangular GNB is formed at 550 K whereas hexagonal GNB is formed at 600 K ( Fig. 2 ). However, we observed that these hexagonal nanobubbles are not nucleated from as-grown triangle bubbles but proceed from a unique blister which acts as the 'epicentre' for the rippling of graphene ( Fig. 2 ) along six directions, as observed in Fig. 1e-f . With increasing reaction time, the hexagonal GNBs grow in size from 2.7, 4.6, 5.4 to 8.1 nm, corresponding to the incorporation of 7, 13, 19 and 37 blisters, as shown in Fig. 1 and Supplementary Fig. S1 . Because the delamination process is thermally activated, the shape and size of the GNB can now be controlled by the annealing temperature and the dosage of oxygen on the Moiré reaction breadboard. Strain-induced pseudo-magnetic field in GNBs Atomic-resolution STM images of the nanobubbles reveal that a triangular lattice is present in highly strained GNBs ( Fig. 3 ), whereas the centre of the relatively smooth GNB shows the typical six-fold symmetry structure. The local electronic structure of Moiré blisters and GNBs is investigated by scanning tunnelling spectroscopy (STS). Individual GNBs exhibit a series of peaks in the STS spectra ( Fig. 1i ), while only one weak peak at −0.43±0.04 eV attributable to the ruthenium substrate is observed in the STS spectrum of the graphene blister ( Supplementary Fig. S2 ) [12] , [21] , [22] . High-resolution STM imaging did not reveal structural defects such as pentagon–heptagon pairs, vacancies or grain boundaries in the lattices of the GNBs ( Fig. 3 ; Supplementary Figs S1 , S3 ; Supplementary Methods ). In addition, the GNBs do not show defects-related signatures in STS data, such as the strong resonance state due to point defects on graphene [23] or tip-height dependence of peak positions associated with the charging of defect states [9] . Therefore, we can rule out the possibility that the observed peaks in the STS spectra are defect-related. The origin of these peaks are most likely associated with Landau levels (LLs) due to strain-induced pseudo-magnetic field, as has been reported previously for GNB observed on graphene grown on Pt [9] . 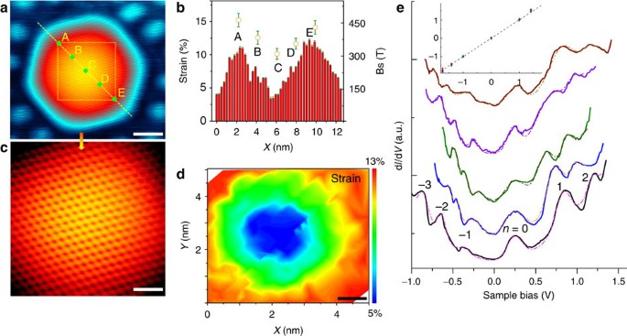Figure 3: STM images and strain mapping of a hexagonal GNB. (a) STM image of a hexagonal GNB. (b) A histogram of experimentally determined local strains along the dashed-line inaand the corresponding pseudo-magnetic field derived from the energy levels in dI/dVspectra shown in (e). (c) Magnified view of the area marked by the square in (a) with its corresponding strain map shown in (d,e), Sequence of five dI/dVspectra taken at A–E points (solid lines ine: black (A), blue (B), olive (C), violet (D), wine (E); dash-lines ine: Gaussian fitting) along a line across a hexagonal GNB shown in (a). Inset of (e): normalized peak energyfor Landau-energy peaks (n=−3,±2,±1,0) observed on A–E points of hexagonal GNB ina, which follow the expected scaling behaviour from the equation in the text (black, red, blue, magenta, olive sets corresponding to normalized peak energy in STS curves of A–E, respectively). The scale bars in (a,c,d) are 2, 1, 1 nm, respectively. Tunnelling parameters (a,c)V=0.2 V,I=0.4 nA. The relativistic nature of massless Dirac particles gives rise to unusual LLs energy sequence, which shows the square-root dependence in both field and level index [9] , [24] : Figure 3: STM images and strain mapping of a hexagonal GNB. ( a ) STM image of a hexagonal GNB. ( b ) A histogram of experimentally determined local strains along the dashed-line in a and the corresponding pseudo-magnetic field derived from the energy levels in d I/ d V spectra shown in ( e ). ( c ) Magnified view of the area marked by the square in ( a ) with its corresponding strain map shown in ( d , e ), Sequence of five d I /d V spectra taken at A–E points (solid lines in e : black (A), blue (B), olive (C), violet (D), wine (E); dash-lines in e : Gaussian fitting) along a line across a hexagonal GNB shown in ( a ). Inset of ( e ): normalized peak energy for Landau-energy peaks ( n =−3,±2,±1,0) observed on A–E points of hexagonal GNB in a , which follow the expected scaling behaviour from the equation in the text (black, red, blue, magenta, olive sets corresponding to normalized peak energy in STS curves of A–E, respectively). The scale bars in ( a , c , d ) are 2, 1, 1 nm, respectively. Tunnelling parameters ( a , c ) V =0.2 V, I =0.4 nA. Full size image where E n is the n th Landau energy with respect to the Fermi level, B S is the pseudo-magnetic field, v F is the Fermi velocity. From equation (1), the LL energy in graphene scales according to E/B 1/2 and the Dirac point ( E D ) is coincident with n =0 state, where E D is derived to be 0.23±0.02 eV from the STS data recorded on a GNB. The shift of Dirac point above Fermi energy indicates a hole-doping effect, possibly from the trapped oxygen species inside the nanobubble [20] . For a GNB with characteristic dimension of l =4 nm and h =0.52 nm ( Fig. 3 ), a spatial dependence of strain-induced B S can be extracted from the position of the LL peak indexed as ' n =1'. Figure 3b shows that a relatively uniform B S of between 300 T to 360 T was generated across the central region of the bubble, and the field increases to 460 T at the edges. A plot of the normalized energy , compiled from five equally spaced positions of GNB shows that the peaks with level index n =−3,−2,−1,0,1,2 follow the expected scaling behaviour for LLs in graphene (inset of Fig. 3e ). To correlate B S with strain, the local strains in GNB are calculated from the changes in C–C bond distances in the graphene lattice ( Supplementary Figs S4 –8 and Supplementary Methods ). Figure 3b shows a histogram of the experimentally determined local strains along a distance of 12 nm in the hexagonally shaped GNB whereas Fig. 3d shows the strain map in the area shown in Fig. 3c . It can be seen that the strain field is not uniform and has an approximately hexagonal symmetry. The strain increases from 3 to 5% in the centre regions to 10–13% at the edges of GNB, which agrees well with the spatial dependence of strain-induced pseudo-magnetic field. We also examined a series of GNBs with different sizes and corrugations. The d I/ d V spectra with their corresponding Gaussian fits are displayed in Fig. 1i and Supplementary Fig. S1 , respectively. The pseudo-magnetic field derived from the LLs-related peaks is in the range 240 T to 600 T ( Supplementary Fig. S1 ). Defect-engineered Ru surface for the controllable growth of GNBs One intriguing observation is that, once a GNB is synthesized at high temperatures and is allowed to cool to room temperature, its size does not increase with a second oxidation reaction. For example, we did not see a triangular nanobubble evolving into a hexagonal one. Very often, a second-stage annealing at a higher temperature causes the bubbles to 'burst' instead, leaving behind a triangular or hexagonal hole ( Fig. 4 ) at 650 K (<etching temperature reported). Regular array of these holes on graphene can form antidots lattice that have been predicted to generate spin qubits [25] , [26] . One explanation for the formation of a hole is that, once the GNB is allowed to cool down, the edges are coupled intimately to the oxidized ruthenium substrate during its contraction and relaxation. At a second stage of oxidative heating, the graphene edges are nicked by a catalytic reaction involving the oxidized Ru(0001) surface to produce CO/CO 2 in the presence of oxygen [27] . Once a hole is formed, oxidative etching of graphene through the edges of the hole is facile owing to the high reactivity of the unsaturated carbon atoms at the edges. Subsequently, these triangular and hexagonal anti-dots grow in size from several nm to several hundred nm with annealing time ( Fig. 4a–c ). The average size of the anti-dots shows a linear dependence with reaction time indicating that the etching process is controlled by oxidation kinetics [19] , [28] . STM imaging of the anti-dot, as shown in Fig. 4e , reveals the presence of a (2×2)-O overlayer on Ru(0001) with a lattice constant of 0.54 nm and O coverage of 0.25 ( Fig. 4d–e and Supplementary Fig. S9 ). These results open up another route for using graphene anti-dots to modify the electronic properties of graphene [25] , [26] . 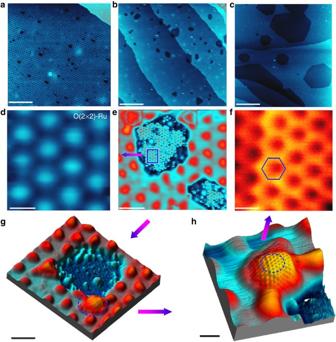Figure 4: The formation of geometric etched antidot at 650 K after the 'burst' of a GNB. (a–c), The evolution of the anti-dot generated in the graphene lattice with different annealing time. The scale bars in (a–c) are 20, 40, 150 nm, respectively. (d–e), Oxidized Ru surface, O(2×2) adlayer in the anti-dot. (d), The magnified view of Ru oxide lattice The scale bars in (d–e) are 0.4, 3 nm, respectively. (f–h), Atomic-resolved image of GNBs in the periphery of the anti-dot reveal that the less strained region (the centre part is relatively flat as marked by blue circle inh) shows the typical six-fold symmetry in (f), while the triangular pattern is present in highly strained region (The slope of the GNB in h). The scale bars in (f–h) are 0.25, 3, 1 nm, respectively Tunnelling parameters (a–c,g)V=1.0 V,I=0.1 nA; (d–e)V=1.0 V,I=1.0 nA; (f, h)V=0.2 V,I=0.4 nA. Figure 4: The formation of geometric etched antidot at 650 K after the 'burst' of a GNB. ( a – c ), The evolution of the anti-dot generated in the graphene lattice with different annealing time. The scale bars in ( a – c ) are 20, 40, 150 nm, respectively. ( d – e ), Oxidized Ru surface, O(2×2) adlayer in the anti-dot. ( d ), The magnified view of Ru oxide lattice The scale bars in ( d – e ) are 0.4, 3 nm, respectively. ( f – h ), Atomic-resolved image of GNBs in the periphery of the anti-dot reveal that the less strained region (the centre part is relatively flat as marked by blue circle in h ) shows the typical six-fold symmetry in ( f ), while the triangular pattern is present in highly strained region (The slope of the GNB in h). The scale bars in ( f – h ) are 0.25, 3, 1 nm, respectively Tunnelling parameters ( a – c , g ) V =1.0 V, I =0.1 nA; ( d – e ) V =1.0 V, I =1.0 nA; ( f, h ) V =0.2 V, I =0.4 nA. Full size image Why does the GNB emerge randomly on the surface? When we examined the spatial distribution of the GNBs on the graphene surface, it was observed that the GNBs frequently emerged at sites next to irregularities on the Moiré pattern (see, for example, the 'dark' areas in Fig. 5 ). When these irregular Moiré patterns were carefully imaged, we did not find any point defects such as pentagon–heptagon pairs or mono- or multi-vacancies ( Supplementary Fig. S10 ). Therefore, we deduce that these 'defects' (that is missing blisters) on the Moiré pattern are due to irregularities at the interface between graphene and the Ru(0001) substrate, which translates into angular distortions and translational domains on graphene, as shown in Supplementary Fig. S10 . STM imaging of the Ru(0001) lattice reveals occasional mono- or multi-vacancies. It can be anticipated that graphene growing over these defects will subsequently have irregularities on its Moiré pattern. More importantly, the defects on Ru(0001) may act as O incorporation site that initiates the growth of surface oxide. Such vacancies are known to exhibit high catalytic activity, because the dissociation of molecular oxygen and the activation energy for O incorporation at these sites is considerably lower than that for bulk oxide formation [29] . 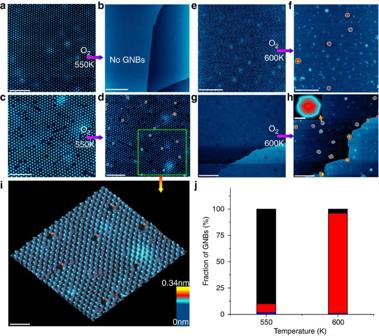Figure 5: STM images showing various shapes, sizes and densities of GNBs. (a–h), The density of GNBs increases with the density of irregularities on the Moiré pattern of graphene on Ru(0001). (a–b), At 550 K and O2pressure of 1.5×10−7mbar for 10 min, no GNBs were observed in 1 μm2of graphene with a perfect Moiré pattern. The scale bars in (a,b) are 20, 200 nm, respectively. (c–d), Under the same conditions, triangular GNBs were achieved with a density of (1±0.2)×105per μm−2, when surface vacancies on Ru(0001) were intentionally created with a density of (1.5±0.3)×105per μm−2. (e–h), At 600 K, the density of hexagonal GNBs is (0.8±0.2)×105per μm−2, correlating closely with the density of Ru surface vacancies of (1.5±0.3)×105per μm−2. The scale bars in (c–d) are 20 nm, and in (e–h) are 30 nm (the scale bar in insert ofhis 3 nm). (i), Magnified view of the marked region in (d) shows the triangular GNBs. The scale bars in (i) is 10 nm. (j), Histogram of the distribution of GNBs with different shapes at different annealing temperatures (black: triangle GNB; red: hexagonal GNB; blue: trapezoid GNB). Tunnelling parameters (a–i)V=1.0 V,I=0.1 nA. Figure 5: STM images showing various shapes, sizes and densities of GNBs. ( a – h ), The density of GNBs increases with the density of irregularities on the Moiré pattern of graphene on Ru(0001). ( a – b ), At 550 K and O 2 pressure of 1.5×10 −7 mbar for 10 min, no GNBs were observed in 1 μm 2 of graphene with a perfect Moiré pattern. The scale bars in ( a , b ) are 20, 200 nm, respectively. ( c – d ), Under the same conditions, triangular GNBs were achieved with a density of (1±0.2)×10 5 per μm −2 , when surface vacancies on Ru(0001) were intentionally created with a density of (1.5±0.3)×10 5 per μm −2 . ( e – h ), At 600 K, the density of hexagonal GNBs is (0.8±0.2)×10 5 per μm −2 , correlating closely with the density of Ru surface vacancies of (1.5±0.3)×10 5 per μm −2 . The scale bars in ( c – d ) are 20 nm, and in ( e – h ) are 30 nm (the scale bar in insert of h is 3 nm). ( i ), Magnified view of the marked region in ( d ) shows the triangular GNBs. The scale bars in ( i ) is 10 nm. ( j ), Histogram of the distribution of GNBs with different shapes at different annealing temperatures (black: triangle GNB; red: hexagonal GNB; blue: trapezoid GNB). Tunnelling parameters ( a – i ) V =1.0 V, I =0.1 nA. Full size image To verify the hypothesis that defect sites act as seeds for the growth of GNBs, we intentionally created surface defects by ion sputtering (500 eV, 0.5 μA) ( Supplementary Fig. S11 ). A high-quality graphene region with perfect Moiré pattern was used as a control during the same condition of O 2 exposure. Indeed, there were no GNBs detected at the defect-free graphene region with the perfect ordering of blisters ( Fig. 5a-b ). However, triangular GNBs with a density of (1±0.2)×10 5 per μm 2 ( Fig. 5d, i ) were observed at the graphene sample with irregular Moiré superstructure. The density of the GNBs agrees well with the density of the surface vacancies on Ru(0001) of (1.5±0.3)×10 5 per μm 2 at 550 K ( Supplementary Fig. S11 ). Similarly, the density of hexagonal GNBs increases from (2±0.2)×10 4 per μm −2 to (0.8±0.2)×10 5 per μm −2 ( Fig. 5e–h ) when the density of Ru surface vacancies is increased from (5±0.2)×10 4 per μm −2 to (1.5±0.3)×10 5 per μm −2 at 600 K ( Supplementary Fig. S11 ). Therefore, we found a direct correlation between the density and spatial distribution of GNBs and the location of subsurface defects. In conclusion, we have demonstrated a systematic approach for the fabrication of geometrically well-defined GNBs using the graphene Moiré superstructure as the reaction 'breadboard'. The growth of the GNBs is achieved by the controlled sintering of periodic surface blisters using an oxidative delamination process. The size and shape of the GNBs and its associated strain-induced pseudo-magnetic field can be controlled by pressure, reaction time or temperature during the oxidation. The premise of using substrate defect engineering on the graphene Moiré 'breadboard' as a means to control the density and distribution of GNBs has also been demonstrated, pointing to the exciting possibility of using these techniques to fabricate GNBs in the desired channel region in graphene transistors. Graphene nanobubbles growth and methods The experiments were performed in an ultrahigh-vacuum chamber with a base pressure of 2×10 −10 mbar. The clean Ru(0001) surface was prepared by repeated cycles of 1 keV-accelerated argon ion sputtering at room temperature with argon pressure of 1×10 −5 mbar. This was followed by annealing in an O 2 pressure of 2×10 −7 mbar at 1,000 K and subsequent flashing to 1,600 K by e-beam heating. To create surface vacancies, the as-prepared Ru(0001) was intentionally exposed to a flux of low-energy argon-ion beam (500 eV, 0.5 μA) for 2 min or 10 min. Ethylene gas (purity 99.99%) at a partial pressure of 2.5×10 −7 mbar was onto the Ru(0001) surface decorated with surface vacancies, and the substrate was annealed at 800–1,000 K to grow extended graphene overlayer. To generate the GNB, the graphene sample which was heated to 550–600 K was exposed to molecular oxygen with partial pressure of 1×10 −7 –2.5×10 −7 mbar for 10–16 min. Scanning tunnelling microscopy and STS measurement The ultrahigh-vacuum-STM employed is a SPECS STM 150 Aarhus unit with the Nanonis (SPECS) SPM control system. STM images were recorded in the constant current mode at sample temperatures of 298 or 100 K (liquid-N 2 cooling). In addition to STM topographic images, the STS data were taken at 100 K, using standard lock-in techniques by adding a modulation voltage 20–50 mV with a frequency of 2.4 kHz. How to cite this article: Lu, J. et al . Transforming moiré blisters into geometric graphene nano-bubbles. Nat. Commun. 3:823 doi: 10.1038/ncomms1818 (2012).